The role of allyl ammonium salts in palladium-catalyzed cascade reactions towards the synthesis of spiro-fused heterocycles There is a continuous need for designing new and improved synthetic methods aiming at minimizing reaction steps while increasing molecular complexity. In this respect, catalytic, one-pot cascade methodologies constitute an ideal tool for the construction of complex molecules with high chemo-, regio-, and stereoselectivity. Herein, we describe two general and efficient cascade procedures for the synthesis of spiro-fused heterocylces. This transformation combines selective nucleophilic substitution (S N 2′), palladium-catalyzed Heck and C–H activation reactions in a cascade manner. The use of allylic ammonium salts and specific Pd catalysts are key to the success of the transformations. The synthetic utility of these methodologies is showcased by the preparation of 48 spiro-fused dihydrobenzofuranes and indolines including a variety of fluorinated derivatives. The development of novel chemical transformations increasing molecular complexity enables significant innovation potential in life and material sciences. In this respect, catalytic cascade or domino processes offer strong impetus for new methodology developments [1] , [2] , [3] . Compared to traditional consecutive procedures, they permit several practical advantages: In addition to improved step-economy, waste generation from multiple iterations of reaction, workup, and purification procedures are minimized. Consequently, diverse and complex organic molecules can be assembled not only in a faster, but also more sustainable way. Since their discovery in the 1970s and 80s [4] , [5] , [6] , [7] , [8] , palladium-catalyzed C–C bond forming reactions have become the most popular homogeneous catalytic processes in organic chemistry and industrial fine chemical synthesis [9] , [10] , [11] , [12] . Their ability to form (stereo)selectively carbon-carbon bonds under mild conditions made them “a true power tool for organic synthesis” [13] . Specifically, the intramolecular Heck reaction provides an entry to useful palladium complexes with quaternary carbon centers as intermediates (Fig. 1b , I – 2 ), which can be further valorized to a multitude of valuable building blocks [14] , [15] , [16] , [17] , [18] . Notably, the combination of this reaction with C–H activation processes has also been studied, giving access to structurally unique spiro compounds [19] , [20] , [21] , [22] , [23] , [24] , [25] , [26] , [27] , [28] , [29] , [30] , [31] , which possess interesting biological activities (Fig. 1c ) [32] , [33] , [34] , [35] , [36] , [37] , [38] . However, the necessity of pre-synthesized starting materials in the existing methods limits the full exploitation of this elegant concept and is often tedious. In our quest for the development of new cascade methodologies, we had the idea to provide a more facile entry to this class of compounds by combining three (or four) palladium-catalyzed coupling processes, namely Tsuji–Trost and Heck reactions followed by selective C–H activation (and alkyne insertion) to assemble complex organic molecules from easily available substrates (Fig. 1 ). Fig. 1: Concepts. a Previous work: palladium-catalyzed intramolecular cyclization for the synthesis of spiroheterocycles. b This work: palladium-catalyzed allylic substitution/Heck/C–H activation(/alkyne) cascade processes. c Selected examples of related bio-active spiro compounds. Full size image Herein, we describe our recent efforts to establish a palladium-catalyzed allylic substitution/Heck/C–H activation(/alkyne) cascade processes for the synthesis of spiro-fused heterocycles. Key challenges of such processes are obviously the compatibility of the well-matched reactant partners [39] , the required conditions of the individual reactions, the development of a general catalyst system able to promote all three (or four) transformations efficiently, and to achieve the needed high chemo-selectivity, regio-selectivity, and stereoselectivity throughout all elementary steps. Reaction development Recently, Lautens, Schoenebeck and co-workers reported the synthesis of spiro-fused heterocycles through an intramolecular Heck/C–H activation sequence using specific alkene-tethered aryl iodides (Fig. 1a ) [40] , [41] , [42] . Regarding the starting materials, those substrates might be preferably prepared through an initial palladium-catalyzed Tsuji-Trost allylation of 2-halophenols, which would provide a more efficient and step-economic way [43] , [44] , [45] . Following this initial idea, we investigated the coupling of 2-iodophenol ( 1a ) with 2-phenylallyl acetate ( 2a ) in the presence of PdBr 2 / L1 (Fig. 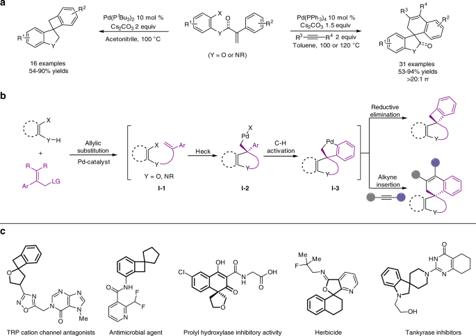Fig. 1: Concepts. aPrevious work: palladium-catalyzed intramolecular cyclization for the synthesis of spiroheterocycles.bThis work: palladium-catalyzed allylic substitution/Heck/C–H activation(/alkyne) cascade processes.cSelected examples of related bio-active spiro compounds. 2a ) and various other palladium catalysts (for details see Supplementary Information, Supplementary Table 1 ). Unfortunately, in no case the desired spiro-fused product 4a was observed and no conversion took place. Similar results were obtained when the tert -butyl (2-phenylallyl) carbonate ( 2b ) was used instead of 2a . When more reactive 2-phenylallyl bromide 2c was introduced, only the alkene-tethered aryl iodide 3a was isolated in 73% yield instead of product 4a . To improve the reactivity of the starting material further on, other allylic leaving groups were considered. In this respect, allylic ammonium salts, which have been largely neglected in intermolecular palladium-catalyzed allylic substitutions, attracted our attention [39] , [46] , [47] . This class of compounds are in general highly stable and can be conveniently prepared from a variety of amines. Surprisingly, testing 2d in the presence of the PdBr 2 / L1 catalyst, the desired cascade process took place and product 4b was obtained in 87% isolated yield! This means that each individual step proceeds with an efficiency of at least 95%. At this point, it should be mentioned that allylic ammonium salts are also known to undergo direct S N 2-substitution or S N 2’-substitution reactions under basic conditions [48] , [49] , [50] . To understand whether the first reaction step is really palladium-catalyzed, 2d was treated with 1a in the presence of 1 equiv. of base. Interestingly, the allyl aryl ether 3b was obtained in high yield (95%). Subsequent reaction in the presence of our regular palladium catalyst led to full consumption of 3b , providing the desired spiro-benzocyclobutane 4b in 87% yield (Fig. 2b ). Obviously, applying substrate 2d does not allow to distinguish between S N 2-mechanism and S N 2’-mechanism in the first reaction step due to its symmetry. Based on the actual interest in fluorinated building blocks [51] , [52] , [53] , the gem -difluorinated allylic ammonium salt 2e [39] was reacted with 2-iodophenol, which gave product 3c in 99% yield and excellent regioselectivity. Again, the following palladium-catalyzed steps took place smoothly and provided 4c in high yield (80%). Similarly, the direct conversion of 2e proceeded efficiently to give 4c in 83% isolated yield (Fig. 2a , entry 5). It should be noted that related fluorinated heterocycles in general cannot be easily prepared [54] and that to the best of our knowledge no example of such spiro compounds has been reported yet. 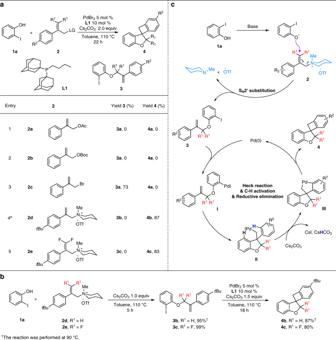Fig. 2: Constructing molecular complexity: spiro-fused heterocycles from simple starting materials. aPreliminary results show the importance of ammonium salts as the partners of the nucleophile.bControl experiments shown that the allylic aryl ether3was formed in situ as important intermediate during the cascade procedure.cA SN2’ substitution process was proposed for the first reaction step, followed by sequence palladium-catalyzed Heck reaction/C–H activation/Pd reductive elimination to provide the target product4. Apart from 2e , other related ammonium salts 2f – 2i underwent similar coupling processes to provide the desired product 4c in slight lower yield (62–75%) (for details see Supplementary Information, Supplementary Table 2 ). Fig. 2: Constructing molecular complexity: spiro-fused heterocycles from simple starting materials. a Preliminary results show the importance of ammonium salts as the partners of the nucleophile. b Control experiments shown that the allylic aryl ether 3 was formed in situ as important intermediate during the cascade procedure. c A S N 2’ substitution process was proposed for the first reaction step, followed by sequence palladium-catalyzed Heck reaction/C–H activation/Pd reductive elimination to provide the target product 4 . Full size image To obtain optimal results, an extensive evaluation of the reaction conditions of the model systems was performed (for details see Supplementary Information, Supplementary Tables 1 – 9 ) and revealed three significant points: (1) The catalyst system is crucial in this cascade process and only in the presence of sterically hindered and electron-rich diadamantyl phosphines such as L1 , the desired product was obtained in high yield. (2) Cs 2 CO 3 and toluene were independently identified as the most effective base and solvent, which nearly doubled the product yield compared to other common bases and solvents. (3) In addition, the concentrations of substrates are decisive. Using an equimolar amount of both substrates led to the best result while an excess of either ammonium salt or aryl halide considerably decreased the yield of 4 . Based on all these observations, a plausible mechanism for the formation of benzocyclobutane derivative 4 is proposed in Fig. 2c : Initially, 2-iodophenol 1 and ammonium salt 2 underwent a base mediated S N 2’ allylic substitution in a highly regioselective manner. To further confirm the S N 2’ route, deuterium substituted ammonium salt was tested, details see Supplementary Information, Supplementary Fig. 1 . Next, intramolecular palladium-catalyzed Heck reaction of the in situ generated compound 3 followed by site-selective C–H activation forms the spiropalladacycle III . Final reductive elimination regenerates the palladium species and produces the desired product [40] . Noteworthily, this novel cascade reaction is a rare example of a domino process involving S N 2´ substitution with subsequent metal-catalyzed transformations [55] , [56] . Scope for the formation of spiro-fused benzocyclobutene derivatives With the optimized reaction conditions in hand, the general feasibility of this approach was examined. As shown in Fig. 3 , allylic ammonium salts with different substituents in 3-position including H, F, CF 3 , directly afforded 4b – 4e in all cases in good to high isolated yields. For disubstituted substrate 2j with –F and –CF 3 substituents in 3-position, high diastereoselectivity for two adjacent quaternary carbon centers was obtained ( 4e , 71%). Next, the reaction of gem -difluorinated allylic ammonium salts 2k – 2u with aryl halides 1a – 1o (for details see Supplementary Information, Supplementary Fig. 2 ) was investigated. Most of the ammonium salts were conveniently obtained from commercially available phenylboronic acid and vinyl bromides via Suzuki reaction, base-mediated amination, and final N -methylation [39] . With regard to the cascade reaction, both electron-donating groups including alkyl, aryl, alkoxy and aryloxy and electron-withdrawing groups including fluoro and chloro were perfectly compatible with the conditions, and the corresponding products 4f – 4l were obtained in 53 − 86% yield. The molecular structure of these highly strained 5,4-spirocycles was unambiguously confirmed by X-ray crystal structure analysis of 4f . Both diphenylamino-substituted and trimethylsilyl-substituted spiro compounds 4m and 4n were successfully formed in high yield. Furthermore, dibenzofuran-derived ammonium salt underwent the cascade process, leading to the construction of the heterocycle-embedded tetracyclic framework 4o in 60% yield. Gratifyingly, the more complex derivative 4p containing two spiro-fused benzocyclobutanes was smoothly generated in 51% yield via a consecutive two-fold cascade process using the corresponding bis-ammonium salt as the reagent. Fig. 3: Palladium-catalyzed cascade reaction of ammonium salts with aryl halides. Standard reaction conditions: 1 (0.2 mmol), 2 (0.2 mmol), Cs 2 CO 3 (0.4 mmol), PdBr 2 (0.01 mmol), L1 (0.02 mmol), toluene (2.5 mL), the reaction mixture was performed at 110 °C under argon atmosphere for 22 h, isolated yield, the diastereoselectivity of 4e , 4p , and 4ac was determined by crude 19 F NMR analyses. † The reaction mixture was performed at 90 °C. ‡ 1 mol% PdBr 2 and 2 mol% L1 were used. § 10 mol% PdBr 2 and 20 mol% L1 were used. ¶ 1 (0.2 mmol), 2 (0.1 mmol) were used. # 2 mol% PdBr 2 and 4 mol% L1 were used. Full size image Next, we explored the scope of our methodology with respect to the aryl halide coupling partner. In addition to 2-iodophenols 1a - 1l , 2-bromophenol 1m , 2-chlorophenol 1n , and 2-iodoaniline 1o were also investigated. The latter case highlights the possibility to construct 3-spiro-indolines, specifically 2-fluorinated indolines ( 4ad and 4ae ), which are of interest as natural products and pharmaceutical molecules [57] , [58] . As depicted in Fig. 3 , several different aryl halides gave the expected tetracyclic products under the standard conditions. Interestingly, considering the three-step cascade, these transformations proceeded in good to excellent yields with either electron-rich or electron-deficient substituents. Notably, substrates containing heteroarenes, such as the quinoline derivative 1k , provided the N , O -fused heterocycle 4ab in 60% yield. Moreover, the L -tyrosine derived product 4ac was obtained by a concise cascade transformation (dr = 1:1). Three-component spirocyclization reaction Considering the versatility of the in-situ-generated palladacycles III [16] , [26] , [27] , subsequent functionalization including carbene and alkyne insertion should allow for the efficient construction of other classes of novel spiro compounds [29] , [30] , [41] , [42] . To demonstrate this synthetic potential, we performed the reaction of 1a and 2e with two equiv. of an additional unsymmetrical alkyne 5a (ethyl 3-phenyl-propynoate). Indeed, the envisioned cascade process combining S N 2’ substitution, palladium-catalyzed Heck/C–H activation and final alkyne insertion provided in a straightforward manner only one regioisomer of the respective 6,5-spirocycles 6 (regioselectivity: >20:1). Under standard conditions, the desired product 6a was obtained in 73% yield; however, in this case the highly reactive palladacycle III also underwent minor reductive elimination and the 5,4-spirocycle 4c was detected in 14% yield. Pleasantly, increasing substrate concentration in the presence of the extended ligand L3 provided exclusively 6a in high yield (85% isolated yield; for a brief evaluation of reaction conditions see Supplementary Information, Supplementary Table 10 ). The generality of this second three-component cascade procedure is shown by variation of five aryl iodides, nine ammonium salts and six alkynes (Fig. 4 ). In all cases, the domino reaction proceeded smoothly with valuable substituents and functional groups, including alkoxy, aryloxy, halide, silyl, and amino, giving the corresponding products 6a – 6h in good to high yields with excellent regioselectivities. 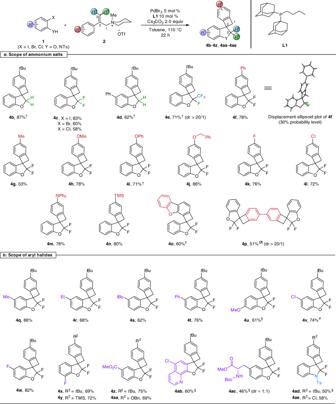Fig. 3: Palladium-catalyzed cascade reaction of ammonium salts with aryl halides. Standard reaction conditions:1(0.2 mmol),2(0.2 mmol), Cs2CO3(0.4 mmol), PdBr2(0.01 mmol),L1(0.02 mmol), toluene (2.5 mL), the reaction mixture was performed at 110 °C under argon atmosphere for 22 h, isolated yield, the diastereoselectivity of4e,4p, and4acwas determined by crude19F NMR analyses.†The reaction mixture was performed at 90 °C.‡1 mol% PdBr2and 2 mol%L1were used.§10 mol% PdBr2and 20 mol%L1were used.¶1(0.2 mmol),2(0.1 mmol) were used.#2 mol% PdBr2and 4 mol%L1were used. 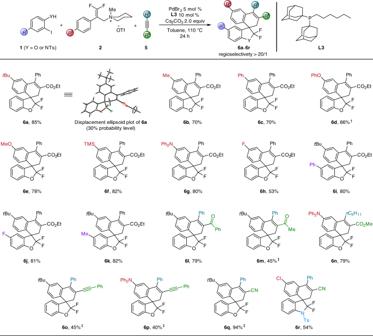Fig. 4: Palladium-catalyzed three-component cascade spriocyclizations. Standard reaction conditions:1(0.2 mmol),2(0.2 mmol),5(0.4 mmol), Cs2CO3(0.4 mmol), PdBr2(0.01 mmol),L3(0.02 mmol), toluene (1.0 mL), the reaction mixture was stirred at 110 °C under argon atmosphere for 24 h, isolated yield, the regioselectivity of6was determined by crude19F NMR analyses.†2 mol% PdBr2and 4 mol%L3were used.‡10 mol% PdBr2and 20 mol%L3were used. The molecular structure of 6a was confirmed by X-ray crystallography. Substituents on the phenyl ring of aryl iodide displayed only a minor influence on the reactivity and provided 6i – 6k in high yields. Notably, various unsymmetrical alkynes with different substituents on the triple bond afforded 6l – 6q with excellent degrees of both chemoselectivities and regioselectivities. For example, internal alkynes bearing −COPh, −COCH 3 , and −CO 2 Me substituents gave the corresponding products 6l – 6n in 79%, 45 and 79% isolated yield, respectively. It is worthy to note that 3-phenyl-2-propynenitrile and 1,3-diynes were compatible in this transformation, affording 6o – 6q in 40–94% isolated yield. Finally, the construction of 3-spiro-indoline 6r was also achieved in 54% yield. Fig. 4: Palladium-catalyzed three-component cascade spriocyclizations. Standard reaction conditions: 1 (0.2 mmol), 2 (0.2 mmol), 5 (0.4 mmol), Cs 2 CO 3 (0.4 mmol), PdBr 2 (0.01 mmol), L3 (0.02 mmol), toluene (1.0 mL), the reaction mixture was stirred at 110 °C under argon atmosphere for 24 h, isolated yield, the regioselectivity of 6 was determined by crude 19 F NMR analyses. † 2 mol% PdBr 2 and 4 mol% L3 were used. ‡ 10 mol% PdBr 2 and 20 mol% L3 were used. Full size image In summary, we have developed two efficient cascade processes involving allylic substitution (via S N 2’-mechanism), palladium-catalyzed Heck, remote C–H activation, and reductive elimination or alkyne insertion for the straightforward synthesis of 5,4-spiroheterocycles and 6,5-spiroheterocycles in good to high yields with excellent selectivities. Crucial for the success of these transformations is the use of specifically activated allylic substrates (ammonium salts) in combination with special PdBr 2 /AlkylPAd 2 catalytic systems. Under optimal conditions diverse (fluorinated) spiro-dihydrobenzofurans and spiro-indolines are achieved in an unprecedented fast and step-economic way, without need for purification of intermediates. We believe these methodologies demonstrate the potential of catalytic cascade processes for a straightforward increase of molecular complexity of simple and easily available aryl halides. General procedure for the preparation of spiro-fused benzocyclobutanes 4 To a 25 ml oven-dried pressure tube equipped with a magnetic stir bar were added 2-halophenol or aniline 1 (0.2 mmol), ammonium salt 2 (0.2 mmol), Cs 2 CO 3 (130 mg, 0.4 mmol), PdBr 2 (2.7 mg, 0.01 mmol), L1 (7.2 mg, 0.02 mmol), and then degassed toluene (2.5 mL) was introduced under argon atmosphere. The sealed pressure tube was heated and stirred at 110 °C for 22 h. The reaction mixture was allowed cooling to room temperature, diluted with ethyl acetate (10 ml), and filtered through a short pad of celite eluting with ethyl acetate (3 × 10 ml). After evaporation, the residue was purified by chromatography on basic aluminum oxide (It is worthy to note that the 2-fluorinated product can only be separated without decomposition using basic aluminum oxide) to afford the desired product 4 . General procedure for the preparation of spiro-fused dihydronaphthalenes 6 To a 25 ml oven-dried pressure tube equipped with a magnetic stir bar were added 2-halophenol or aniline 1 (0.2 mmol), ammonium salt 2 (0.2 mmol), alkyne 5 (0.4 mmol), Cs 2 CO 3 (130 mg, 0.4 mmol), PdBr 2 (2.7 mg, 0.01 mmol), L3 (7.7 mg, 0.02 mmol), and then degassed toluene (1 ml) was introduced under argon atmosphere. The sealed pressure tube was heated and stirred at 110 °C for 24 h. The reaction mixture was allowed cooling to room temperature, diluted with ethyl acetate (10 ml), and filtered through a short pad of celite eluting with ethyl acetate (3 × 10 ml). After evaporation, the residue was purified by chromatography on basic aluminum oxide (It is worthy to note that the 2-fluorinated product can only be separated without decomposition using basic aluminum oxide) to afford the desired product 6 .